Glycogen synthase kinase 3β ubiquitination by TRAF6 regulates TLR3-mediated pro-inflammatory cytokine production TRAF6 is critical for the production of inflammatory cytokines in various TLR-mediated signalling pathways. However, it is poorly understood how TRAF6 regulates TLR3 responses. Here we demonstrate that GSK3β interacts with TRAF6 and positively regulates the TLR3-mediated signalling. Suppression of GSK3β expression or its kinase activity drastically reduces the production of inflammatory cytokines and the induction of c-Fos by decreasing ERK and p38 phosphorylation. GSK3β physically associates with TRAF6 in a TLR3 ligand poly I:C-dependent manner. TRAF6 is determined to be a direct E3 ligase for GSK3β, and TRAF6-mediated GSK3β ubiquitination is essential for poly I:C-dependent cytokine production by promoting the TLR3 adaptor protein TRIF-assembled signalling complex. Toll-like receptors (TLRs) comprise a class of conserved type I transmembrane pattern recognition receptors [1] that recognize pathogen-associated molecular patterns and play a critical role in the host cell defence against microbial pathogens [2] . The recognition of pathogen-associated molecular patterns by TLRs activates multiple pathways that mediate immune responses to produce immune mediators, including pro-inflammatory cytokines, chemokines and type I interferons (IFNs) [2] , [3] , [4] . In particular, TLR3 signalling through the recognition of double-stranded RNA is crucial for antiviral responses [5] , [6] , [7] . Upon ligand binding to TLR3, the sole cytoplasmic adaptor molecule toll-interleukin 1 receptor homology-domain-containing adapter-inducing interferon-β (TRIF) is recruited to the TLR signalling complex [8] , [9] . The TLR3–TRIF signalling complex further triggers the recruitment of downstream signalling molecules, including tumour necrosis factor (TNF) receptor-associated factor 3 (TRAF3) [10] , TRAF6 (ref. 11 ) and receptor-interacting protein 1 (RIP1) [12] , which lead to the activation of IFN regulatory factor 3 (IRF3) [13] , activator protein 1 (AP1) [14] and nuclear factor-kappa B (NF-κB) [15] . While the TLR3-mediated signalling pathways in type I IFN production have been well explored, little is known about their regulatory mechanisms in pro-inflammatory cytokine production. Glycogen synthase kinase 3 (GSK3) is a highly conserved serine/threonine kinase that was originally identified as a regulator of glycogen metabolism [16] . Two highly related isoforms of GSK3 exist, GSK3α and GSK3β, and they are ubiquitously expressed in mammalian tissues [17] . Although both isoforms share similar structural features, they are not functionally identical [18] . GSK3β plays crucial roles in various signal pathways that regulate multiple cellular functions, including metabolism, cell proliferation, differentiation and development [19] , [20] , [21] . GSK3β is also involved in diverse TLR signalling [22] , [23] . For example, GSK3β has been identified as a key mediator of pro-inflammatory cytokine production, including interleukin (IL)-6, TNF-α, IL-12p40, IL-1β and IFN-γ, and anti-inflammatory cytokine IL-10 production by regulating CREB activity in Myd88-dependent TLR pathways [24] , [25] . In addition, GSK3β differentially regulates the production of lipopolysaccharide (LPS)-induced IL-Iβ and the endogenous IL-1 receptor antagonist through ERK activity [26] . Another study demonstrated that GSK3β regulated IFN-γ-induced signal transducer and activator of transcription 3 (STAT3) activity and was required for the synergistic action of LPS and IFN-γ on IL-6 cytokine production [27] . Although these studies clearly document the importance of GSK3β in TLR-mediated cytokine production, little is known about the role of GSK3β in TLR3 signalling. In this report, we show that GSK3β is essential for TLR3-mediated ERK and p38 activation, c-Fos induction and pro-inflammatory cytokine production. We also find that GSK3β undergoes a lysine (K)-63 chain ubiquitination, which is important for assembling the TRIF signalling complex for TLR3 signalling. Our findings provide insights into the molecular mechanisms underlying the regulatory function of GSK3β in TLR3-mediated pro-inflammatory cytokine production. GSK3β regulates TLR3-triggered innate immune response Previous reports demonstrated the crucial roles of GSK3β in TLR-mediated pro-inflammatory cytokine production through the myeloid differentiation factor 88 (MyD88)-dependent pathway [24] , [25] , [28] , [29] . However, how GSK3β regulates TLR3 signalling through a TRIF-dependent pathway [8] , [9] , [30] remains unclear. To examine the involvement of GSK3β in TLR3 signalling, we generated the RAW264.7 macrophage cell line stably expressing a GSK3β-specific short hairpin RNA (shRNA) ( Fig. 1a ). In real-time PCR analysis, the messenger RNA (mRNA) levels of pro-inflammatory cytokines, including IL-6, TNF-α, interferon-γ-inducible protein 10 (IP-10) and IL-12, greatly decreased in the GSK3β knockdown RAW264.7 cells compared with the levels in control cells after a TLR3 ligand, poly I:C, stimulation ( Fig. 1a ). In parallel with suppression of mRNAs, knockdown of GSK3β led to a decrease TLR3-mediated IL-6 and TNF-α protein production ( Supplementary Fig. 1a ). The differential effects of GSK3β inhibition on production of pro- and anti-inflammatory cytokines after TLR2, TLR4, TLR5 and TLR9 stimulation have been reported [24] . Unlike those TLRs, TLR3 stimulation in GSK3β knockdown RAW264.7 cells showed a decrease in anti-inflammatory cytokine IL-10 production in mRNA and protein levels ( Fig. 1a ; Supplementary Fig. 1b ). Although both GSK3α and GSK3β were phosphorylated in response to poly I:C ( Fig. 1b ), overexpression of GSK3β but not its homologue GSK3α significantly elevated IL-6 and TNF-α mRNA expression in a dose-dependent manner ( Fig. 1c ). We next used a GSK3 inhibitor SB216763 to determine whether the kinase activity of GSK3 was responsible for inflammatory cytokine production. GSK3 inhibition with SB216763 resulted in a substantial reduction in IL-6, TNF-α and IL-10 levels compared with the levels in untreated cells after poly I:C stimulation ( Fig. 1d ). Importantly, poly I:C-induced mRNA and protein expression levels of IL-6, TNF-α and IL-10 were impaired in Gsk3b −/− mouse embryonic fibroblasts (MEFs) ( Fig. 1e ; Supplementary Fig. 2 ). Reconstitution with GSK3β but not GSK3α or the kinase inactive GSK3β (K85A) mutant into Gsk3b −/− MEFs by transient overexpression restored the poly I:C-induced mRNA expression of IL-6, TNF-α and IL-10 ( Fig. 1e ). Consistently, silencing of GSK3β but not GSK3α in bone marrow-derived macrophages (BMDMs) inhibited induction of inflammatory cytokines, including IL-6, TNF-α and IL-10 ( Supplementary Fig. 3a–c ). Thus, these results suggest that GSK3β positively regulates TLR3-mediated inflammatory cytokine production and that the kinase activity of GSK3β is required for its role in poly I:C-induced cytokine production. 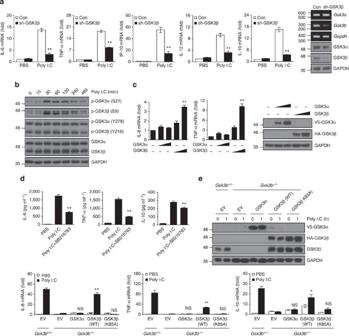Figure 1: GSK3β but not GSK3α is involved in TLR3-mediated pro-inflammatory cytokine production. (a) RAW264.7 cells stably expressing control shRNA (Con) or GSK3β-specific shRNA (sh-GSK3β) were stimulated with 10 μg ml−1poly I:C for 1 h. Levels of IL-6, TNF-α, IP-10, IL-12 and IL-10 mRNA were determined by real-time PCR analysis, and the values were normalized to β-actin mRNA expression. GSK3β knockdown was confirmed by reverse transcription-PCR and western blotting. (b) BMDMs were treated with 10 μg ml−1poly I:C for the indicated time points. Whole-cell lysates were immunoblotted with antibodies to the molecules along the right margin. (c) HEK293-TLR3 cells were transiently transfected with V5-GSK3α or HA-GSK3β plasmids. Levels of IL-6 and TNF-α mRNA were determined as described ina. Expression of the transduced proteins was detected by western blotting with anti-V5 (for GSK3α) and anti-HA (for GSK3β). (d) BMDMs were preincubated for 1 h with or without 10 μM SB216763 and stimulated with or without 10 μg ml−1poly I:C for 20 h. Levels of IL-6, TNF-α and IL-10 in culture supernatants were determined by enzyme-linked immunosorbent assay. (e)Gsk3b−/−MEFs were transiently transfected with V5-GSK3α, HA-GSK3β (WT) or GSK3β (K85A) plasmids, and cells were stimulated with 10 μg ml−1poly I:C for 1 h. Levels of IL-6, TNF-α and IL-10 mRNA were determined as described ina. Expression of the transduced proteins was detected by western blotting as described inc. Data are presented as the mean±s.d. from at least three independent experiments. Statistical analyses were calculated using the Student’st-test (*P<0.05; **P<0.01; NS, not significant). Figure 1: GSK3β but not GSK3α is involved in TLR3-mediated pro-inflammatory cytokine production. ( a ) RAW264.7 cells stably expressing control shRNA (Con) or GSK3β-specific shRNA (sh-GSK3β) were stimulated with 10 μg ml −1 poly I:C for 1 h. Levels of IL-6, TNF-α, IP-10, IL-12 and IL-10 mRNA were determined by real-time PCR analysis, and the values were normalized to β-actin mRNA expression. GSK3β knockdown was confirmed by reverse transcription-PCR and western blotting. ( b ) BMDMs were treated with 10 μg ml −1 poly I:C for the indicated time points. Whole-cell lysates were immunoblotted with antibodies to the molecules along the right margin. ( c ) HEK293-TLR3 cells were transiently transfected with V5-GSK3α or HA-GSK3β plasmids. Levels of IL-6 and TNF-α mRNA were determined as described in a . Expression of the transduced proteins was detected by western blotting with anti-V5 (for GSK3α) and anti-HA (for GSK3β). ( d ) BMDMs were preincubated for 1 h with or without 10 μM SB216763 and stimulated with or without 10 μg ml −1 poly I:C for 20 h. Levels of IL-6, TNF-α and IL-10 in culture supernatants were determined by enzyme-linked immunosorbent assay. ( e ) Gsk3b −/− MEFs were transiently transfected with V5-GSK3α, HA-GSK3β (WT) or GSK3β (K85A) plasmids, and cells were stimulated with 10 μg ml −1 poly I:C for 1 h. Levels of IL-6, TNF-α and IL-10 mRNA were determined as described in a . Expression of the transduced proteins was detected by western blotting as described in c . Data are presented as the mean±s.d. from at least three independent experiments. Statistical analyses were calculated using the Student’s t -test (* P <0.05; ** P <0.01; NS, not significant). Full size image GSK3β is involved in retinoic acid-inducible gene 1-like receptor (RLR)-mediated antiviral response [31] . Since TLR- and RLR-mediated signalling pathways share a number of components, we examined whether GSK3β is also involved in poly I:C-stimulated IRF3 activation and IFN-β induction. We found that poly I:C stimulation induced increased phosphorylation of TBK1, a kinase responsible for phosphorylating IRF3 after poly I:C stimulation, in wild-type MEFs but not Gsk3b −/− MEFs ( Supplementary Fig. 4a ). Consistently, deficiency of GSK3β markedly inhibited poly I:C-induced IRF3 phosphorylation and nuclear translocation ( Supplementary Fig. 4a,b ) as well as dimerization of IRF3 ( Supplementary Fig. 4c ). Consistently, neither Gsk3b −/− MEFs nor GSK3β knockdown RAW264.7 cells showed significant induction of IFN-β upon poly I:C stimulation ( Supplementary Fig. 4d ). We further confirmed that silencing of GSK3β but not GSK3α in BMDMs inhibited IFN-β induction significantly ( Supplementary Fig. 4e ). It is interesting to note that GSK3 inhibition with SB216763 did not alter poly I:C-induced IFN-β mRNA expression ( Supplementary Fig. 4f ), suggesting that the effect of GSK3β on TLR3-mediated IFN-β induction is independent of its kinase activity. Together, these data indicate that GSK3β is required for TLR3-mediated IRF3 activation and the type I IFN-β induction. GSK3β regulates TLR3-mediated ERK and p38 activation The mitogen-activated protein kinases (MAPKs) and the NF-κB signalling pathways are important for inflammatory cytokine production in TLR signalling [32] , [33] , [34] . To examine whether GSK3β regulates MAPKs and NF-κB activation in TLR3 signalling, we analysed the phosphorylation levels of ERK, p38, JNK and NF-κB p65 in GSK3β knockdown RAW264.7 cells. As shown in Fig. 2a , GSK3β knockdown markedly decreased poly I:C-induced ERK and p38 phosphorylation levels, whereas there were no significant differences in the phosphorylation levels of JNK and NF-κB p65. Similar results were observed in BMDMs silenced by short interfering RNA (siRNAs) specific for GSK3β. Although knockdown of both forms of GSK3 appears to delay poly I:C-induced IκB-α degradation, silencing of GSK3β but not GSK3α significantly reduced poly I:C-induced ERK and p38 activation ( Supplementary Fig. 5 ). These results were further confirmed in Gsk3b −/− MEFs. Phosphorylation levels of ERK and p38 but not JNK, IKKα/β, IκB-α and NF-κB p65 were significantly decreased in Gsk3b −/− MEFs compared with the levels in Gsk3b +/+ MEFs ( Fig. 2b ; Supplementary Fig. 6a ). In reporter assays, knockdown or overexpression of GSK3β did not affect poly I:C-induced NF-κB activation, further suggesting that GSK3β is not involved in TLR3-mediated NF-κB signalling ( Supplementary Fig. 6b,c ). Because a TRIF-dependent pathway is also involved in TLR4 signalling [35] , [36] , we examined the effects of GSK3β on LPS-induced MAPKs and NF-κB p65 phosphorylation levels. Interestingly, the GSK3β knockdown decreased LPS-induced phosphorylation levels of p38 and JNK but not ERK and NF-κB p65 ( Fig. 2c ). In contrast, there were no significant differences between GSK3β knockdown RAW264.7 and control cells after a TLR2 ligand, Pam3CSK4, stimulation ( Fig. 2d ). It should be noted that Pam3CSK4-induced MAPKs and NF-κB p65 phosphorylation is mediated by a Myd88-dependent, but not a TRIF-dependent, pathway. Thus, these data indicate that GSK3β regulates ERK and p38 MAPK activation in TRIF-dependent TLR3 signalling. 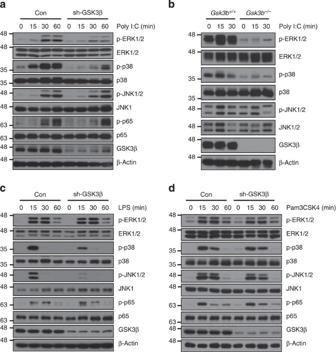Figure 2: GSK3β regulates poly I:C-mediated ERK and p38 activation. (a) Western blotting of the phosphorylation of the MAPKs ERK, p38 and JNK and NF-κB p65 in poly I:C-stimulated RAW264.7 cells stably expressing control shRNA (Con) or GSK3β-specific shRNA (sh-GSK3β). (b) Western blotting of ERK, p38 and JNK phosphorylation inGsk3b+/+andGsk3b−/−MEFs stimulated with 10 μg ml−1poly I:C. (c,d) As ina, except that the cells were stimulated with 100 ng ml−1LPS (c) or 100 ng ml−1Pam3CSK4 (d) as indicated. Data are representative of two or three independent experiments. Figure 2: GSK3β regulates poly I:C-mediated ERK and p38 activation. ( a ) Western blotting of the phosphorylation of the MAPKs ERK, p38 and JNK and NF-κB p65 in poly I:C-stimulated RAW264.7 cells stably expressing control shRNA (Con) or GSK3β-specific shRNA (sh-GSK3β). ( b ) Western blotting of ERK, p38 and JNK phosphorylation in Gsk3b +/+ and Gsk3b −/− MEFs stimulated with 10 μg ml −1 poly I:C. ( c , d ) As in a , except that the cells were stimulated with 100 ng ml −1 LPS ( c ) or 100 ng ml −1 Pam3CSK4 ( d ) as indicated. Data are representative of two or three independent experiments. Full size image GSK3β regulates expression of c-Fos through ERK and p38 AP1, comprising Jun, c-Fos and ATF2, is activated in response to TLR stimulation and regulates the production of pro-inflammatory cytokines [14] , [37] , [38] . To identify transcription factors regulated by the TLR3–GSK3β axis, we separated the cytosolic and nuclear fractions of GSK3β knockdown RAW264.7 cells after poly I:C stimulation. Interestingly, the c-Fos protein levels in the nuclear fraction appeared drastically reduced in GSK3β knockdown RAW264.7 cells compared with the levels in control cells, whereas nuclear ATF2, c-Jun and NF-κB p65 protein levels were comparable in both cell types ( Fig. 3a ; Supplementary Fig. 7 ), suggesting that GSK3β regulates TLR3-mediated c-Fos expression but not ATF2, c-Jun and NF-κB p65. Consistently, treatment with the GSK3 inhibitor SB216763 or silencing of GSK3β but not GSK3α significantly reduced c-Fos mRNA or protein after TLR3 stimulation ( Fig. 3b,c ), whereas overexpression of GSK3β but not GSK3α produced a substantial increase in c-Fos mRNAs ( Supplementary Fig. 8 ). Reconstitution of GSK3β but not GSK3α or the kinase inactive GSK3β (K85A) mutant into Gsk3b −/− MEFs by transient transfection restored poly I:C-induced c-Fos mRNA expression ( Fig. 3d ). Moreover, the knockdown of c-Fos markedly reduced poly I:C-induced IL-6 and TNF-α expression ( Supplementary Fig. 9 ), confirming the importance of GSK3β-mediated c-Fos expression in TLR3 signalling. 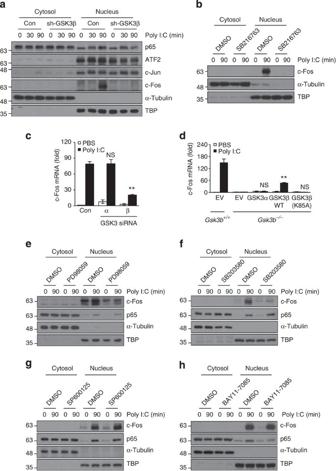Figure 3: GSK3β regulates poly I:C-mediated c-Fos induction through the ERK and p38 pathways. (a) RAW264.7 cells stably expressing control shRNA (Con) or GSK3β-specific shRNA (sh-GSK3β) were stimulated with 10 μg ml−1poly I:C for the indicated time points. Cells were separated into cytosolic and nuclear fractions, and the protein levels of p65, ATF2, c-Jun and c-Fos were determined by western blotting. α-tubulin and TBP served as markers for the cytosolic and nuclear fractions, respectively. (b) As ina, except that the cells were preincubated with dimethylsulphoxide or 10 μM SB216763 for 1 h and then stimulated with 10 μg ml−1poly I:C for 90 min. Cytosolic and nuclear c-Fos levels were determined by western blotting. (c) BMDMs transfected with 20 nM control siRNAs (Con) or GSK3α- or GSK3β-specific siRNAs were stimulated with 10 μg ml−1poly I:C for 1 h. Levels of c-Fos mRNA were determined by real-time PCR. (d) As inc, except thatGsk3b+/+andGsk3b−/−MEFs were transiently transfected with V5-GSK3α, HA-GSK3β (WT) or GSK3β (K85A) plasmids. (e–h) As inb, except that the cells were preincubated with 10 μM PD98059 (e), 10 μM SB203580 (f), 25 μM SP600125 (g) or 10 μM BAY 11-7085 (h) for 1 h and then stimulated with 10 μg ml−1poly I:C for 90 min. Cytosolic and nuclear c-Fos and p65 protein levels were determined by western blotting. Data are presented as the mean±s.d. from at least three independent experiments. Statistical analyses were calculated using the Student’st-test (**P<0.01; NS, not significant). Figure 3: GSK3β regulates poly I:C-mediated c-Fos induction through the ERK and p38 pathways. ( a ) RAW264.7 cells stably expressing control shRNA (Con) or GSK3β-specific shRNA (sh-GSK3β) were stimulated with 10 μg ml −1 poly I:C for the indicated time points. Cells were separated into cytosolic and nuclear fractions, and the protein levels of p65, ATF2, c-Jun and c-Fos were determined by western blotting. α-tubulin and TBP served as markers for the cytosolic and nuclear fractions, respectively. ( b ) As in a , except that the cells were preincubated with dimethylsulphoxide or 10 μM SB216763 for 1 h and then stimulated with 10 μg ml −1 poly I:C for 90 min. Cytosolic and nuclear c-Fos levels were determined by western blotting. ( c ) BMDMs transfected with 20 nM control siRNAs (Con) or GSK3α- or GSK3β-specific siRNAs were stimulated with 10 μg ml −1 poly I:C for 1 h. Levels of c-Fos mRNA were determined by real-time PCR. ( d ) As in c , except that Gsk3b +/+ and Gsk3b −/− MEFs were transiently transfected with V5-GSK3α, HA-GSK3β (WT) or GSK3β (K85A) plasmids. ( e – h ) As in b , except that the cells were preincubated with 10 μM PD98059 ( e ), 10 μM SB203580 ( f ), 25 μM SP600125 ( g ) or 10 μM BAY 11-7085 ( h ) for 1 h and then stimulated with 10 μg ml −1 poly I:C for 90 min. Cytosolic and nuclear c-Fos and p65 protein levels were determined by western blotting. Data are presented as the mean±s.d. from at least three independent experiments. Statistical analyses were calculated using the Student’s t -test ( ** P <0.01; NS, not significant). Full size image Considering the defects in ERK and p38 MAPK signalling in GSK3β knockdown RAW264.7 cells and Gsk3b −/− MEFs ( Fig. 2a,b ), it is likely that poly I:C-mediated ERK and p38 MAPK activation regulates c-Fos expression. To test this hypothesis, we assessed c-Fos expression in the presence of the ERK inhibitor PD98059, the p38 inhibitor SB203580, the JNK inhibitor SP600125 or the NF-κB inhibitor BAY 11-7085. Expectedly, ERK or p38 inhibition markedly reduced poly I:C-induced c-Fos protein levels compared with the levels of the dimethylsulphoxide control ( Fig. 3e,f ). In contrast, nuclear c-Fos expression was not affected by the inhibition of JNK or NF-κB ( Fig. 3g,h ). Together, these data indicate that GSK3β regulates poly I:C-induced c-Fos expression via ERK and p38 activation. GSK3β is required for TLR3 signalling complex formation Upon poly I:C stimulation, activated TLR3 initiates the interaction of TRIF with TRAF6, transforming growth factor β-activated kinase 1 (TAK1) and RIP1 to activate MAPKs and NF-κB signalling cascades [11] , [12] , [39] . Specifically, the TRIF–TRAF6–TAK1 axis is important for the activation of MAPKs, which in turn leads to AP1 activation [34] , [39] , [40] . To examine how GSK3β regulates MAPKs in TLR3 signalling, we first determined the roles of GSK3β in forming the TLR3 signalling complex following poly I:C stimulation in Gsk3b −/− MEFs. In control cells, poly I:C stimulation induced recruitment of TRIF, RIP1, TRAF6, TAK1, TAK1-binding protein 1 (TAB1), TAB2 and GSK3β to TLR3, which persisted for at least 30 min ( Fig. 4 ). Interestingly, GSK3β deficiency prevented the recruitment of TRAF6, TAK1, TAB1 and TAB2 to TLR3, but had no effect on the recruitment of TRIF and RIP1. Consistently, silencing of GSK3β in RAW264.7 macrophages impaired the poly I:C-triggered formation of the TLR3 signalling complex containing TRAF6, TAK1, TAB1 and TAB2 ( Supplementary Fig. 10a ). Notably, pretreatment with the GSK3 inhibitor SB216763 in BMDMs also blocked the formation of the poly I:C-induced TLR3 signalling complex ( Supplementary Fig. 10b ). Thus, these results suggest that GSK3β is important for recruiting the TRAF6–TAK1–TAB1–TAB2 complex to TLR3. 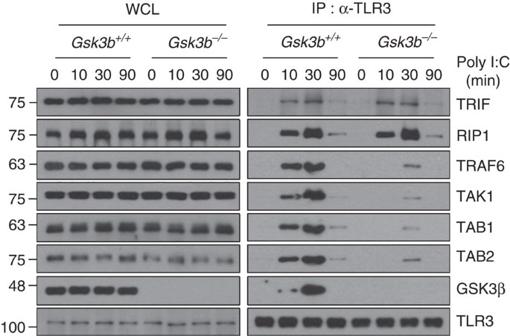Figure 4: GSK3β is required for the recruitment of the TRAF6–TAK1–TAB1–TAB2 complex to TLR3. Gsk3b+/+andGsk3b−/−MEFs were stimulated with 10 μg ml−1poly I:C for 10 min and subjected to immunoprecipitation with an anti-TLR3 antibody. TRIF, RIP1, TRAF6, TAK1, TAB1, TAB2 and GSK3β protein levels from whole-cell lysates (WCL) and TLR3 immunocomplexes (IP: α-TLR3) were determined by western blotting. Data are representative of two independent experiments. Figure 4: GSK3β is required for the recruitment of the TRAF6–TAK1–TAB1–TAB2 complex to TLR3. Gsk3b +/+ and Gsk3b −/− MEFs were stimulated with 10 μg ml −1 poly I:C for 10 min and subjected to immunoprecipitation with an anti-TLR3 antibody. TRIF, RIP1, TRAF6, TAK1, TAB1, TAB2 and GSK3β protein levels from whole-cell lysates (WCL) and TLR3 immunocomplexes (IP: α-TLR3) were determined by western blotting. Data are representative of two independent experiments. Full size image GSK3β interacts with TRAF6 and TAK1 To further explore the regulatory mechanisms of GSK3β in TLR3 signalling, we investigated the interaction of GSK3β with TRAF6 and TAK1. TAK1, a MAP3K family member [41] , is a critical transducer molecule downstream of TRAF6, and the TRAF6–TAK1 axis activates MAPKs in TLR signalling [2] , [42] , [43] . We first examined by co-immunoprecipitation experiments whether GSK3β associates with TRAF6 or TAK1 upon poly I:C stimulation in BMDMS. The results indicated that GSK3β indeed associates with TRAF6 and/or TAK1 under physiological conditions ( Fig. 5a ). We next examined whether TRAF6, GSK3β and TAK1 bind to one another, forming a ternary complex. To examine this binding, HEK293T cells were transfected with a Flag-TRAF6 construct with or without a Myc-TAK1 or HA-GSK3β construct. We observed that Flag-TRAF6 co-immunoprecipitated with Myc-TAK1 and HA-GSK3β, indicating that TRAF6 forms a ternary complex with GSK3β and TAK1 ( Fig. 5b ). Similarly, we further confirmed the association of GSK3β with TRAF6 and TAK1 as well as TAK1 with TRAF6 and GSK3β by cotransfection studies in mammalian cells ( Supplementary Fig. 11a,b ). Notably, deletion of GSK3β prevented association of TRAF6 with TAK1 upon poly I:C stimulation ( Fig. 5c ). We also investigated the interaction of GSK3β with RIP1, an essential mediator of TLR3-induced NF-κB activation [12] . Unlike TRAF6 and TAK1, however, RIP1 did not interact with GSK3β ( Supplementary Fig. 12a,b ), further confirming that GSK3β is not involved in NF-κB signalling mediated by the TLR3–TRIF–RIP1 axis. 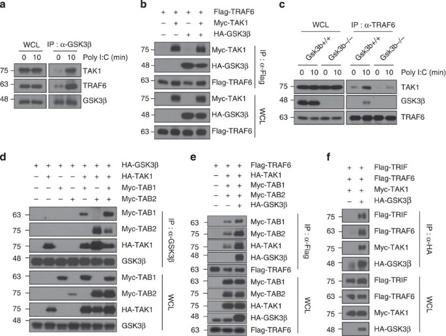Figure 5: GSK3β associates with TRAF6, TAK1 and TRIF. (a) BMDMs were stimulated with 10 μg ml−1poly I:C for 10 min and subjected to immunoprecipitation with an anti-GSK3β antibody. TRAF6 and TAK1 protein levels from whole-cell lysates (WCL) and TLR3 immunocomplexes (IP: α-GSK3β) were determined by western blotting. (b) GSK3β formed a ternary complex with TRAF6 and TAK1. HEK293T cells were transfected with the indicated combinations of expression plasmids. Co-imunoprecipitations were performed with anti-Flag antibody followed by western blotting with the indicated antibodies. The expression levels of the transfected plasmids were confirmed by western blot analysis of whole-cell lysates. (c) As inFig. 4b, except that whole-cell lysates were immunoprecipitated with anti-TRAF6 antibody followed by western blotting as indicated. (d) GSK3β associated with TAB1 and TAB2 through TAK1. These experiments were performed as described inb. (e) TRAF6 associated with TAB1, TAB2, TAK1 and GSK3β. The experiments were performed as described inb. (f) GSK3β associates with TRIF, TRAF6 and TAK1. The experiments were performed as described inb. Data are representative of two or three independent experiments. Figure 5: GSK3β associates with TRAF6, TAK1 and TRIF. ( a ) BMDMs were stimulated with 10 μg ml −1 poly I:C for 10 min and subjected to immunoprecipitation with an anti-GSK3β antibody. TRAF6 and TAK1 protein levels from whole-cell lysates (WCL) and TLR3 immunocomplexes (IP: α-GSK3β) were determined by western blotting. ( b ) GSK3β formed a ternary complex with TRAF6 and TAK1. HEK293T cells were transfected with the indicated combinations of expression plasmids. Co-imunoprecipitations were performed with anti-Flag antibody followed by western blotting with the indicated antibodies. The expression levels of the transfected plasmids were confirmed by western blot analysis of whole-cell lysates. ( c ) As in Fig. 4b , except that whole-cell lysates were immunoprecipitated with anti-TRAF6 antibody followed by western blotting as indicated. ( d ) GSK3β associated with TAB1 and TAB2 through TAK1. These experiments were performed as described in b . ( e ) TRAF6 associated with TAB1, TAB2, TAK1 and GSK3β. The experiments were performed as described in b . ( f ) GSK3β associates with TRIF, TRAF6 and TAK1. The experiments were performed as described in b . Data are representative of two or three independent experiments. Full size image TAK1 forms a complex with its adaptor proteins TAB1 and TAB2. TAB2 bridges TRAF6 to TAK1, allowing TAK1 activation [44] , [45] , [46] . We therefore investigated whether GSK3β could associate with TAB1 or TAB2 and affect the formation of the signalling complex containing TRAF6, TAK1, TAB1 and TAB2. In contrast to the GSK3β–TAK1 interaction, there was little association between GSK3β and TAB1 or TAB2 ( Fig. 5d , lanes 3 and 4). However, GSK3β could associate with TAB1 or TAB2 in the presence of TAK1, indicating that the association of GSK3β with TAB1 or TAB2 requires TAK1. Notably, forced expression of GSK3β promotes the association of TRAF6 with the TAK1–TAB1–TAB2 complex ( Fig. 5e , lane 3). Furthermore, overexpressed GSK3β binds to TRIF, TRAF6 and TAK1 as a complex ( Fig. 5f ). Altogether, these results demonstrate that GSK3β could form a TRIF-assembled signalling complex containing TRAF6–TAB1–TAB2–TAK1. TRAF6 is required for ubiquitination of GSK3β Because TRAF6 possesses E3 ubiquitin ligase activity [47] , [48] , [49] , we next questioned whether GSK3β is ubiquitinated by TRAF6 in TLR3 signalling. We first identified the binding regions between TRAF6 and GSK3β. GSK3β interacted with the TRAF6 (289–530) derivative containing just the coiled-coil TRAF-N domain and the conserved TRAF-C domain, whereas the N-terminal ring and zinc-finger domains of TRAF6 spanning amino acids (aa) 1–289 failed to interact with GSK3β ( Supplementary Fig. 13a ). On the other hand, serial deletion constructs of GSK3β revealed that the N-terminal region spanning aa 1–120 is necessary for TRAF6 interaction ( Supplementary Fig. 13b ). We next tested whether GSK3β is ubiquitinated upon poly I:C stimulation in BMDMs and found that poly I:C triggered polyubiquitination of GSK3β ( Fig. 6a ). Furthermore, overexpression of TRAF6 induced GSK3β ubiquitination ( Fig. 6b ). In contrast, the catalytically inactive TRAF6 (C70A) mutant, which has lost its E3 ligase activity, lost the ability to promote GSK3β ubiquitination ( Fig. 6c ). Ubiquitination of GSK3β occurred mainly through K63 linkage ( Supplementary Fig. 14 ). Unlike TRAF6, NEDD4-1 and TRAF3, two E3 ubiquitin ligases that catalyse K63 ubiquitination and function in CD40 and TLR2 signalling, respectively [50] , [51] , did not promoted GSK3β ubiquitination ( Supplementary Fig. 15 ). TRAF6 deficiency markedly decreased ubiquitination of endogenous GSK3β compared with the ubiquitination of wild-type cells upon poly I:C stimulation ( Fig. 6d ). Moreover, TRAF6 induced GSK3β ubiquitination in vitro ( Fig. 6e ). These results suggest that TRAF6 is an E3 ubiquitin ligase for GSK3β. 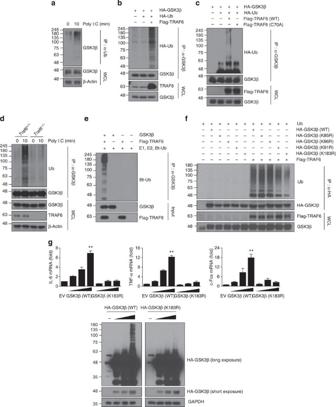Figure 6: TRAF6-mediated GSK3β ubiquitination at lysine 183 is critical for TLR3-dependent cytokine production. (a) BMDMs were stimulated with 10 μg ml−1poly I:C for 10 min and subjected to immunoprecipitation with an anti-Ub antibody followed by western blotting with an anti-GSK3β antibody. (b) HEK293T cells transfected with HA-GSK3β and HA-Ub along with Flag-TRAF6 plasmids were subjected to immunoprecipitation with an anti-GSK3β antibody followed by western blotting with an anti-HA antibody. (c) HEK293T cells were transfected with HA-GSK3β and HA-Ub along with TRAF6 (WT) or TRAF6 (C70A) plasmids. These experiments were performed as described inb. (d)Traf6+/+andTraf6−/−3T3 cells stimulated with 10 μg ml−1poly I:C for 10 min were subjected to immunoprecipitation with an anti-GSK3β antibody followed by western blotting with an anti-Ub antibody. (e) GSK3β proteins were incubated with E1, E2 and biotinylated-Ub (Bt-Ub) in the presence or absence of Flag-TRAF6 proteins forin vitroubiquitination of GSK3β. Ubiquitination of GSK3β was analysed by western blotting with streptavidin-HRP. (f) HEK293T cells transfected with Ub and Flag-TRAF6 along with HA-GSK3β WT or various HA-GSK3β mutants were subjected to immunoprecipitation with an anti-HA antibody followed by western blotting with an anti-Ub antibody. (g) HEK293-TLR3 cells were transiently transfected with GSK3β (WT) or GSK3β (K183R) plasmids. The levels of IL-6, TNF-α and c-Fos mRNA were determined by real-time PCR analysis (top). GSK3β expression levels were confirmed by western blotting with an anti-HA antibody (bottom). A longer exposure of the HA blot shows the presence of ubiquitin ladder. Data are presented as the mean±s.d. from at least three independent experiments. Statistical analyses were calculated using the Student’st-test (**P<0.01). Figure 6: TRAF6-mediated GSK3β ubiquitination at lysine 183 is critical for TLR3-dependent cytokine production. ( a ) BMDMs were stimulated with 10 μg ml −1 poly I:C for 10 min and subjected to immunoprecipitation with an anti-Ub antibody followed by western blotting with an anti-GSK3β antibody. ( b ) HEK293T cells transfected with HA-GSK3β and HA-Ub along with Flag-TRAF6 plasmids were subjected to immunoprecipitation with an anti-GSK3β antibody followed by western blotting with an anti-HA antibody. ( c ) HEK293T cells were transfected with HA-GSK3β and HA-Ub along with TRAF6 (WT) or TRAF6 (C70A) plasmids. These experiments were performed as described in b . ( d ) Traf6 +/+ and Traf6 −/− 3T3 cells stimulated with 10 μg ml −1 poly I:C for 10 min were subjected to immunoprecipitation with an anti-GSK3β antibody followed by western blotting with an anti-Ub antibody. ( e ) GSK3β proteins were incubated with E1, E2 and biotinylated-Ub (Bt-Ub) in the presence or absence of Flag-TRAF6 proteins for in vitro ubiquitination of GSK3β. Ubiquitination of GSK3β was analysed by western blotting with streptavidin-HRP. ( f ) HEK293T cells transfected with Ub and Flag-TRAF6 along with HA-GSK3β WT or various HA-GSK3β mutants were subjected to immunoprecipitation with an anti-HA antibody followed by western blotting with an anti-Ub antibody. ( g ) HEK293-TLR3 cells were transiently transfected with GSK3β (WT) or GSK3β (K183R) plasmids. The levels of IL-6, TNF-α and c-Fos mRNA were determined by real-time PCR analysis (top). GSK3β expression levels were confirmed by western blotting with an anti-HA antibody (bottom). A longer exposure of the HA blot shows the presence of ubiquitin ladder. Data are presented as the mean±s.d. from at least three independent experiments. Statistical analyses were calculated using the Student’s t -test (** P <0.01). Full size image To search for the sites of GSK3β that are responsible for ubiquitination, we generated a series of full-length GSK3β variants containing a lysine residue mutation based on mass spectrometry (MS) analysis ( Supplementary Table 1 ). We mutated K85, K86, K91 or K183 to arginine and then tested the susceptibility of these mutants, when expressed ectopically, to be ubiquitinated by TRAF6. TRAF6-mediated ubiquitination of GSK3β was substantially reduced when with K183R, but not with K85R, K86R or K91R ( Fig. 6f ). Importantly, overexpression of the GSK3β K183R mutant significantly reduced mRNA expression of IL-6 and TNF-α as well as c-Fos in a dose-dependent manner compared with that of the overexpressed wild-type GSK3β ( Fig. 6g ). In similar experiments, reconstitution of GSK3β but not GSK3β (K183R) mutant into Gsk3b −/− MEFs restored the poly I:C-induced IL-6, TNF-α, IL-10 and c-Fos mRNA expression ( Supplementary Fig. 16a,b ) and GSK3β ubiquitination ( Supplementary Fig. 16c ). Because GSK3β (1–120) lacking the K183 residue could bind to TRAF6 ( Supplementary Fig. 13b ), we tested whether GSK3β (1–120) can be ubiquitinated by TRAF6. As expected, GSK3β (1–120) failed to be ubiquitinated by TRAF6 ( Supplementary Fig. 17 ). Interestingly, GSK3β (1–120) could act as a dominant-negative mutant to inhibit poly I:C-induced mRNA expression of IL-6, TNF-α and c-Fos ( Supplementary Fig. 18 ). GSK3β ubiquitination is required for interaction with TRAF6 In our earlier experiments, we showed that GSK3β, TRAF6 and TAK1 bind to one another to form a ternary complex ( Fig. 5b ; Supplementary Fig. 11a,b ) and that GSK3β associates with TRIF, TRAF6 and TAK1 as a complex ( Fig. 5f ). Therefore, we tested whether GSK3β ubiquitination influenced its interaction with TRIF, TRAF6 and TAK1. Overexpression of the GSK3β K183R mutant, which is defective in GSK3β ubiquitination by TRAF6, showed impaired association with TRAF6 compared with the association of wild-type GSK3β ( Fig. 7a ). However, the K183R mutation of GSK3β did not abrogate interactions with TRIF or TAK1 ( Fig. 7b,c ), suggesting that GSK3β ubiquitination by TRAF6 is essential for its interaction with TRAF6. Because either deficiency or a pharmacological inhibition of GSK3β impaired the poly I:C-triggered formation of the TLR3 signalling complex ( Fig. 4 ), we tested whether the GSK3β K183R mutant produced similar effects. Forced expression of the GSK3β ϰ183R mutant markedly decreased the association of GSK3β with TRIF, TRAF6 and TAK1 ( Fig. 7d ; Supplementary Fig. 19 ), as well as the formation of the TRIF-assembled signalling complex containing TRAF6, GSK3β and TAK1 ( Fig. 7e ). Together, our results show that TRAF6-mediated GSK3β ubiquitination is essential for TRAF6 interaction, thereby contributing to the formation of the TRIF–GSK3β–TRAF6–TAK1 complex. 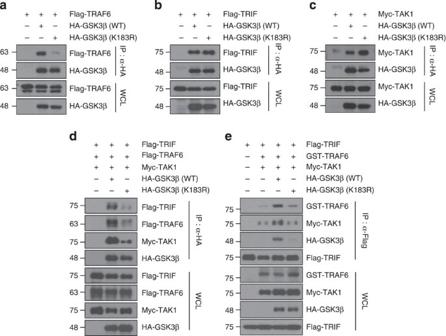Figure 7: Ubiquitination of GSK3β is required for the formation of a signalling complex containing TRIF, TRAF6, TAK1 and GSK3β. (a–c) The GSK3β K183R mutant abrogates the interaction of GSK3β with TRAF6 but not with TRIF or TAK1. HEK293T cells were transfected with the indicated combinations of expression plasmids. Co-imunoprecipitations were performed with an anti-HA antibody followed by western blotting with the indicated antibodies. The expression levels of the transfected plasmids were confirmed by western blotting of whole-cell lysates. (d,e) The GSK3β K183R mutation disrupts the TRIF–GSK3β–TRAF6–TAK1 complex. HEK293T cells were transfected with the indicated combinations of expression plasmids. Co-imunoprecipitations were performed with anti-HA (d) or with anti-Flag (e) antibodies followed by western blotting with the indicated antibodies. The expression levels of the transfected plasmids were confirmed by western blotting of whole-cell lysates. Data are representative of two or three independent experiments. Figure 7: Ubiquitination of GSK3β is required for the formation of a signalling complex containing TRIF, TRAF6, TAK1 and GSK3β. ( a – c ) The GSK3β K183R mutant abrogates the interaction of GSK3β with TRAF6 but not with TRIF or TAK1. HEK293T cells were transfected with the indicated combinations of expression plasmids. Co-imunoprecipitations were performed with an anti-HA antibody followed by western blotting with the indicated antibodies. The expression levels of the transfected plasmids were confirmed by western blotting of whole-cell lysates. ( d , e ) The GSK3β K183R mutation disrupts the TRIF–GSK3β–TRAF6–TAK1 complex. HEK293T cells were transfected with the indicated combinations of expression plasmids. Co-imunoprecipitations were performed with anti-HA ( d ) or with anti-Flag ( e ) antibodies followed by western blotting with the indicated antibodies. The expression levels of the transfected plasmids were confirmed by western blotting of whole-cell lysates. Data are representative of two or three independent experiments. Full size image In general, TLRs that recognize bacteria induce pro-inflammatory cytokines, whereas those TLRs that detect viruses trigger the IFN response [2] , [3] , [4] . These two responses depend on the engagement of the major two adaptor molecules, MyD88 (refs 28 , 29 ) and TRIF [8] , [9] . All TLRs, with the exception of TLR3, signal through the MyD88-dependent pathway [1] , [2] , whereas TRIF-mediated signalling includes TLR3 (refs 6 , 7 ) and TLR4 (refs 35 , 36 ).GSK3β is a crucial regulator in the balance between pro- and anti-inflammatory cytokines in MyD88-dependent TLR signalling [24] , as well as viral-triggered RLR-mediated activation [31] . However, how GSK3β controls TLR3-mediated pro-inflammatory signalling mediated by TRIF, but not by MyD88, is still unknown. We therefore examined whether GSK3β is involved in pro-inflammatory cytokine production in TLR3 signalling and explored the molecuar basis of GSK3β’s role. We found that GSK3β selectively regulated the TLR3-mediated activation of ERK and p38 but not JNK or NF-κB. Notably, the ERK and p38 pathways were required for the induction of c-Fos, which forms the AP1 complex [2] , [14] , [38] . We also found that GSK3β was incorporated into a TLR3-assembled multiprotein complex, and its signalling funtion was regulated by TRAF6-mediated ubiquitination. In the TLR3-assembled signalling complex, GSK3β undergoes polyubiquitination, which is dependent on the E3 ligase activity of TRAF6, and thereby promotes the formation of the TRIF–GSK3β–TRAF6–TAK1 complex. Notably, a ubiquitination-defective GSK3β mutant acts as a dominant-negative form of GSK3β regarding the induction of pro-inflammtory cytokines, as well as c-Fos. The present study establishes an important role for GSK3β in poly I:C-triggered inflammatory cytokine production and provides a mechanistic explanation for how the TRAF6–GSK3β axis selectively regulates TLR3 signalling. In addition, we found that GSK3β in TLR3 signalling had a positive role in regulating the production of TBK1-mediated type I IFN-β. Similar to our results, it was previously shown that GSK3β functions in RLR-mediated IFN-β production by promoting TBK1 and IRF3 activation [31] , suggesting that the IFN-β production triggered by TLR3 and RLRs share a common pathway that converge upon TBK1, which is regulated by GSK3β through its kinase activity-independent mechanism. Among TRAF family members, TRAF3 positively regulates IRF3 and IFN-β response through TRIF interaction [10] , [52] . Therefore, it is likely that the TRAF6–GSK3β axis controls MAPK signalling and c-Fos expression by TLR3, while the TRAF3–GSK3β–TBK1 axis regulates IRF3 activation and IFN-β induction. Indeed, we found that GSK3β interacts with TRAF3 ( Supplementary Fig. 20a ). Furthermore, GSK3β can form a complex containing TRIF, TRAF3 and TBK1 ( Supplementary Fig. 20b ). Interestingly, GSK3β differentially regulates TLR-induced signalling. Our results have demonstrated that GSK3β regulates TLR3- and TLR4-mediated MAPK activation but is not required for TLR2 signalling [53] , [54] , [55] . Because TLR-mediated responses are controlled mainly by the MyD88-dependent pathway [2] , [28] , [29] , which is used by all TLRs except TLR3, and the TRIF-dependent pathway [8] , [9] , [30] , which is used by TLR3 and TLR4 (refs 35 , 36 ), we propose that GSK3β selectively regulates TRIF-dependent MAPK activation. Our results also showed that GSK3β differentially regulates TLR3- and TLR4-mediated MAPKs signalling. GSK3β was required for ERK and p38 pathway activation downstream of TLR3, and for the JNK and p38 pathway activation downstream of TLR4. It is probable that endosomal TRIF signalling complexes downstream of TLR3 and TLR4 are not identical, and differences in their signalling potentials correlate with their ability to selelctively engage GSK3β and thereby dictate downstream MAPK activation. In TRIF-dependent TLR3 signalling, TRIF directly recruits TRAF6 and RIP1, which work cooperatively to activate TAK1, eventually leading to activation of NF-κB and AP1 (refs 11 , 39 , 40 ). In the case of TLR4 stimulation, the initial step of TRIF signalling is mediated through an adaptor TRAM [56] , [57] . Internalized TLR4 recruits TRAF6 to the endosome via TRAM–TRIF [58] , [59] . Consequently, TRAF6 and RIP1 mediate the TRIF-induced activation of MAPKs and NF-κB, respectively [39] , [40] . In this regard, the TRIF-assembled signalling complex of TLR3 or TLR4 formed in different ways, and this may have accounted for the differential regulation of GSK3β in MAPK activation. Although the exact mechanisms of the GSK3β-mediated differential activation of MAPKs in the TLR3 and TLR4 signalling pathways require further investigations, our study suggests that GSK3β selectively regulates TRIF-dependent MAPK activation pathways. Phosphorylation by GSK3β results in activation or inhibition of many its substrates [18] , [20] , [21] . Our results have demonstrated that the kinase activity of GSK3β is required for its ability to induce inflammatory cytokine production. These findings suggest that kinase activity of GSK3β in TLR3–TRIF signalling complex is involved in the cytokine production. Indeed, we found that Ser/Thr phosphorylation of TRAF6 was enhanced in control cells after poly I:C stimulation compared with that in the knockdown of GSK3β ( Supplementary Fig. 21 ), suggesting that TRAF6 might be a candidate among GSK3β substrates. Alternatively, it has been recently reported that Bruton’s tyrosine kinase is required for the production of inflammatory cytokines in TLR3-stimulated macrophages [60] , suggesting that Bruton’s tyrosine kinase acts in TLR3/TRIF signalling. Further studies will be required for characterizing GSK3β substrate(s) in the TLR3–TRIF complex. TRAF6, as an E3 ubiquitin ligase, is known to be a common signalling adaptor for cytokine production in response to various TLR ligands [61] , [62] . TRAF6 can ubiquinate itself on lysine 63, and TRAF6 autoubiquitination in turn recruits mediators for the activation of downstream MAPKs and NF-κB signalling pathways [2] , [48] , [63] . TRAF6 mediates both MyD88-dependent and TRIF-dependent activation of NF-κB and AP1. In MyD88-dependent and TRIF-dependent TLR signalling, ubiquitinated TRAF6 serves as a signalling scaffold to recruit TAK1 via TAB2 and TAB3 (refs 11 , 45 , 46 , 64 ). The TAK1 signalling complex, including TRAF6–TAB2–TAB3–TAB1–TAK1 is subsequently released into the cytosol, where TAK1 activates MAPK cascades [43] , [46] , [64] . Although TRAF6 appears to be a common factor employed by MyD88- and TRIF-dependnent signalling, it is probable that a specific signalling partner, substrate or other signalling protein(s) in each signalling complex is needed for signalling specificity or fine tuning of signalling. In this regard, we have now demonstrated that GSK3β underwent K63 chain ubiquitination. TRAF6 was found to be a direct E3 ligase for GSK3β and was essential for GSK3β ubiquitination, TRIF-assembled signalling complex formation and pro-inflammtory cytokine production upon TLR3 stimulation. This mechanism involves the TLR3-induced assembly of a multiprotein complex containing TRIF, TRAF6, TAB1, TAB2, TAK1 and GSK3β. Complex assembly resulted in TRAF6 autoubiquitination and activation, which led to K63-linked ubiquitination of GSK3β. Ubiquitinated GSK3β promoted a multiprotein-assembled signalling complex, where TAK1 and its subordinate MAPKs are activated. Notably, during IL-1 and receptor activator of nuclear factor-κB ligand signalling, TRAF6 autoubiquitination was dispensable for both interaction with and activation of the TAK1 signalling complex [65] . It has been suggested that TRAF6-mediated K63-linked ubiquitination instead targets relevant protein substrates during activation [63] , [64] . Accordingly, we propose that TRAF6 mediates the K63-linked ubiquitination of GSK3β, which would form a signalling complex sufficient to meet activation thresholds and/or to generate signalling specificity. It should be noted that TRAF6-mediated GSK3β ubiquitination proceeds through a two-stage mechanism. This mechanism involves an initial interaction prior to ubiquitination between TRAF6 and GSK3β. The interaction of TRAF6 (through a coiled-coil TRAF-N domain and a conserved TRAF-C domain) with GSK3β (through a N-terminal region spanning aa 1–120) may lead to K63-linked ubiquitination of GSK3β by E3 ligase activity of TRAF6. We thus propose that GSKβ is a novel TRAF6 substrate downstream of TLR3. The establishment of a regulatory role for GSK3β in TLR3-mediated signalling contributes to the elucidation of the complicated molecular mechanisms of inflammatory and antiviral responses. Cell culture and transfection MEFs from Gsk3b +/+ and Gsk3b −/− mice were kindly provided by Dr J. Woodgett (Ontario Cancer Institute, Toronto, ON, Canada). 3T3 cell lines from Traf6 +/+ and Traf6 −/− mice were established in culture from E14.5 embryos using a standard 3T3 protocol [66] . HEK293-TLR3 stable cell lines were obtained from Dr I.H. Choi (Yonsei University College of Medicine, Seoul, Republic of Korea). Cells were cultured in Dulbecco’s modified Eagle’s medium (DMEM, Hyclone, Logan, UT, USA) supplemented with 10% (v/v) fetal bovine serum (FBS, Hyclone), 100 units ml −1 penicillin (Hyclone) and 100 μg ml −1 streptomycin (Hyclone). Murine BMDMs were obtained from the femurs of 8–10-week-old C57BL/6 male mice. Bone marrow cells were flushed out from the bone marrow cavity, suspended in DMEM supplemented with 20% (v/v) FBS. After 1 day, non-adherent cells were cultured in the presence of 10 ng ml −1 recombinant human macrophage colony-stimulating factor (R&D Systems, Minneapolis, MN, USA). After 7 days, a homogeneous population of adherent macrophages was obtained. To generate the GSK3β knockdown RAW264.7 stable cell lines, non-targeting control and GSK3β shRNA (5′-CATGAAAGTTAGCAGAGATAA-3′) plasmid constructs were purchased from Sigma (St Louis, MO, USA). RAW264.7 cells were transfected with either a non-targeting control or GSK3β shRNA plasmids using a Microporator MP-100 (Invitrogen, Carlsbad, CA, USA) and then selected in DMEM supplemented with 10% (v/v) FBS containing 4 μg ml −1 puromycin (Sigma) for 2 weeks. HEK293T cells and HEK293-TLR3 cells were transfected with the indicated plasmids for 36 h using Lipofectamine 2000 (Invitrogen) according to the manufacturer’s protocol. Non-targeting control siRNA (sc-37007) and c-Fos siRNA (sc-29222) were purchased from Santa Cruz Biotechnology (Santa Cruz, CA, USA). GSK3α siRNA (5′-AAAGCGTCAGTCGGGGCTATGTT-3′) and GSK3β (5′-ACACGAAAGTGATTGGAAATT-3′) siRNA were synthesized by Genolution (Seoul, Republic of Korea). For transient transfection of siRNA, cells were transfected with either a non-targeting control or target-specific siRNA duplexes for 36 h using a Lipofectamine RNAiMAX (Invitrogen) according to the manufacturer’s protocol. Reagents and antibodies TLR3 agonist poly I:C, SB216763, BAY 11-7085, PD98059 and SB203580 were purchased from Sigma. Antibodies specific to phospho-GSK3α/β (S21/S9, 9331, dilution 1:1,000), phospho-ERK (T202/Y204, 4370, dilution 1:1,000), phospho-JNK (T183/185, 9251, dilution 1:1,000), phospho-p38 (T180/Y182, 9215, dilution 1:1,000), phospho-p65 (S536, 3031, dilution 1:1,000), GSK3β (9315, dilution 1:1,000) TAK1 (4505, dilution 1:1,000), ERK (4695, dilution 1:1,000), JNK (9258, dilution 1:1,000), p38 (8690, dilution 1:1,000), p65 (8242, dilution 1:1,000), ATF2 (9226, dilution 1:1,000) and c-Jun (9165, dilution 1:1,000) were purchased from Cell Signaling Technology (Beverly, MA, USA). Antibodies specific to TRAF6 (sc-7221, dilution 1:1,000), c-Fos (sc-7202, dilution 1:1,000), haemagglutinin (HA) (sc-7392, dilution 1:1,000), Myc (sc-40, dilution 1:1,000), glutathione S-transferase (GST) (sc-138, dilution 1:1,000), TBP (sc-204, dilution 1:1,000), ubiquitin (sc-8017, dilution 1:1,000), β-actin (sc-87778, dilution 1:1,000), α-tubulin (sc-58666, dilution 1:1,000) and GAPDH (sc-87724, dilution 1:1,000) were from Santa Cruz Biotechnology. A GSK3α/β-specific antibody (44–610, dilution 1:5,000) was purchased from Invitrogen, and a RIP1-specific antibody (610459, dilution 1:2,000) was purchased from BD Pharmingen (San Diego, CA, USA). A Flag-specific antibody was purchased from Sigma (F3156, dilution 1:5,000), and horseradish peroxidase (HRP)-conjugated secondary antibodies were obtained from Thermo Fisher Scientific (Waltham, MA, USA). Plasmid constructs Wild-type GSK3β plasmid was obtained from Dr J.K. Chung (Seoul National University, Seoul, Republic of Korea). To generate the various GSK3β (K85R, K86R, K91R and K183R) mutants, site-directed mutagenesis was performed by PCR. DNA fragments encoding the GSK3β and various deletion mutants were prepared by PCR and cloned into the pEGFP-N3 and pEBG expression vectors. The wild-type GSK3α plasmid was provided by Dr J. Woodgett. Wild-type and mutant TRAF6, TAB1 and TAB2 plasmids were described previously [65] . The wild-type TAK1 plasmid was a gift from Dr T. Ishitani (Kyushu University, Fukuoka, Japan). Wild-type ubiquitin plasmid was provided by Dr J.H. Seol (Seoul National University), and the wild-type TRIF plasmid was obtained from Dr W.S. Ryu (Yonsei University, Seoul, Republic of Korea). Immunoprecipitation and western blot analysis Cells were washed with cold PBS (Hyclone) and lysed with lysis buffer (50 mM Tris-HCl, pH 8.0, 150 mM NaCl, 0.5% deoxycholate acid, 1% NP-40) containing phosphatase and protease inhibitors. For immunoprecipitation, lysates were incubated with the indicated primary antibodies at 4 °C for 16 h, and were further incubated with protein A-agarose (Millipore, Billerica, MA, USA) at 4 °C for 1 h with gentle shaking. After washing five times with lysis buffer, immunoprecipitated proteins were boiled with 2 × SDS loading buffer, and separated on SDS–polyacrylamide gel electrophoresis (PAGE) and electrophoretically transferred to polyvinylidene difluoride membranes (Millipore). Membranes were blocked with 5% BSA in Tris-buffered saline containing 0.1% Tween-20 and were immunoreacted with the indicated primary antibodies and secondary antibodies conjugated to HRP. Images have been cropped for presentation. Full-size images of all western blots are provided in Supplementary Fig. 22 . Enzyme-linked immunosorbent assay To measure mouse IL-6, TNF-α and IL-10 levels, BMDMs were preincubated with the indicated inhibitors and then stimulated with or without 10 μg ml −1 poly I:C for 20 h. Cell culture supernatants were assessed using ELISA kits from R&D Systems according to the manufacturer’s instructions. Real-time PCR analysis Total RNA was extracted from cells using the TRIzol reagent (Invitrogen) and reverse transcribed to complementary DNA using the Superscript cDNA synthesis kit (Invitrogen) following the manufacturer’s instructions. Real-time PCR analysis was performed using the KAPA SYBR green FAST qPCR kit (Kapa Biosystems, Boston, MA, USA) on an ABI 7300 real-time PCR machine (Applied Biosystems, Foster City, CA). Samples were analysed in triplicate and normalized to β-actin mRNA expression. Primer sequences are listed in Supplementary Table 2 . Cytosolic and nuclear fractionation Cells were lysed with cytosolic extraction buffer (10 mM HEPES, pH 7.4, 10 mM KCl, 1.5 mM MgCl 2 , 0.5 M dithiothreitol, 0.05% NP-40) containing protease inhibitors. After centrifugation at 8,000 r.p.m. for 5 min at 4 °C, supernatants were collected for the cytosolic fraction. Pellets were washed with cytosol extraction buffer and then lysed with nuclear extraction buffer (5 mM HEPES, pH 7.4, 300 mM NaCl, 1.5 mM MgCl 2 , 0.2 mM EDTA, 25% glycerol) containing protease inhibitors. After incubation on ice for 30 min, the nuclear fraction was obtained by centrifugation at 14,000 r.p.m. for 30 min at 4 °C. In vivo ubiquitination assay The in vivo ubiquitination assay was performed as previously described [67] . Briefly, cells were lysed with SDS lysis buffer (50 mM Tris-HCl, pH 6.8, 150 mM NaCl, 10% glycerol, 1% SDS) containing protease inhibitors. After boiling for 5 min, lysates were diluted 10-fold with dilution buffer (10 mM Tris-HCl, pH 8.0, 150 mM NaCl, 2 mM EDTA, 1% Triton X-100) containing protease inhibitors and incubated at 4 °C for 30 min. After centrifugation at 20,000 r.p.m. for 30 min at 4 °C, supernatants were subjected to immunoprecipitation with the indicated antibodies. In vitro ubiquitination assay The GSK3β protein was obtained from Invitrogen (cat # PV3365) and the Flag-TRAF6 protein was purified as previously described [68] . Briefly, HEK293T cells transfected with Flag-TRAF6 for 48 h were lysed in a lysis buffer (10 mM Tris-HCl, pH 7.5, 10 mM NaCl, 1.5 mM MgCl 2 ) containing protease inhibitors and immunoprecipitated with an anti-Flag affinity gel (Sigma) for 16 h at 4 °C. Immunoprecipitates were washed and eluted with 300 μg ml −1 Flag peptide according to the manufacturer’s instructions. The in vitro ubiquitination assay was performed as previously described with minor modifications [67] . Briefly, 5 nM Flag-TRAF6 and 1 μM GSK3β protein were mixed with 100 nM His-E1, 1 μM His-E2 (Ubc13/Mms2) and 2.5 μM Bt-Ub in 50 μM ubiquitination reaction buffer from the ubiquitination kit (Enzo Life Sciences, Farmingdale, NY, USA) according to the manufacturer’s instructions. Samples were subsequently immunoprecipitated with an anti-GSK3β antibody and separated on SDS–PAGE followed by streptavidin conjugated to HRP (Thermo Fisher Scientific). GST pull-down assay Cells were washed with cold PBS and lysed with lysis buffer (20 mM HEPES, pH 7.4, 150 mM NaCl, 150 mM KCl, 10 mM EDTA, 10% glycerol, 1% NP-40) containing phosphatase and protease inhibitors. Whole-cell lysates were incubated with glutathione-sepharose 4B (GE Healthcare, Piscataway, NJ, USA) at 4 °C for 3 h with gentle shaking. After washing three times with lysis buffer, proteins were boiled with 2 × SDS loading buffer. Native PAGE assay For detection of IRF3 dimerization, Gsk3b +/+ and Gsk3b −/− MEFs stimulated with 10 μg ml −1 poly I:C for 1 h were lysed in a lysis buffer (50 mM Tris-HCl, pH 7.5, 150 mM NaCl, 0.5% NP-40) containing protease inhibitors. After centrifugation at 20,000 r.p.m. for 10 min, supernatants were mixed with 2 × native sample buffer (100 mM Tris-Cl, pH 6.8, 30% glycerol and 2% deoxycholate). Gels (7.5%) (without SDS) were pre-run with 25 mM Tris and 192 mM glycine, pH 8.3, with and without 1% deoxycholate in the cathode and anode chamber, respectively, for 1 h at 10 mA and 4 °C. Subsequently, samples were applied to the gel and electrophoresed for ~1 h at 20 mA and 4 °C and transferred to polyvinylidene difluoride membranes (Millipore) for 1 h at 270 mA and 4 °C. Luciferase assay RAW264.7 cells were transiently transfected with pGL3-Basic or pGL3-NF-κB-luc along with pRL-TK-renilla luciferase plasmids. HEK293-null or HEK293-TLR3 cells were transiently transfected with pGL3-NF-κB-luc and pRL-TK-renilla luciferase along with pEGFP-N3 or pEGFP-N3-GSK3β plasmids. After 24 h transfection, cells were stimulated with 10 μg ml −1 poly I:C for 4 h and luciferase activity was measured with the Dual-Luciferase Reporter Assay System (Promega, Madison, WI, USA) according to the manufacturer’s instructions. Samples were analysed in triplicate and normalized to renilla luciferase activity. Mapping of ubiquitination sites on GSK3β For identification of ubiquitination sites on GSK3β, HEK293T cells were transfected with HA-tagged GSK3β expression plasmids for 36 h. Cells were lysed with lysis buffer (20 mM Tris-HCl, pH 7.4, 1% SDS), boiled for 5 min, sonicated and then diluted 10-fold with NP-40 lysis buffer (20 mM Tris-HCl, pH 7.4, 150 mM NaCl, 2 mM EDTA, 1% NP-40). After centrifugation at 15,000 g for 15 min, the lysates were incubated with 120 μl of anti-HA Agarose (Thermo scientific) at 4 °C overnight with rotation. The beads were washed four times with NP-40 lysis buffer and eluted with 2 × SDS–PAGE sample buffer without a reducing agent. HA-GSK3β proteins eluted from the beads were subjected to SDS–PAGE followed by Coomassie Blue staining or western blot analysis. For MS analysis, gel bands from the Coomassie Blue stained-gel were excised and subjected to trypsin digestion and liquid chromatography–MS/MS. MS/MS data were analysed using SEQUEST (Thermo Finnigan, San Jose, CA) software to identify ubiquitin modification with the GG or LRGG remnant tag on lysine residues of GSK3β. Statistical analysis Data are presented as the mean±s.d. from at least three independent experiments. Statistical significance was determined using Student’s t -test. How to cite this article: Ko, R. et al. Glycogen synthase kinase 3β ubiquitination by TRAF6 regulates TLR3-mediated pro-inflammatory cytokine production. Nat. Commun. 6:6765 doi: 10.1038/ncomms7765 (2015).